Photo-mediated selective deconstructive geminal dihalogenation of trisubstituted alkenes Selective deconstructive functionalization of alkenes, other than the well-established olefin metathesis and ozonolysis, to produce densely functionalized molecular scaffolds is highly attractive but challenging. Here we report an efficient photo-mediated deconstructive germinal dihalogenation of carbon-carbon double bonds. A wide range of geminal diiodoalkanes and bromo(iodo)alkanes (>40 examples) are directly prepared from various trisubstituted alkenes, including both cyclic and acyclic olefins. This C=C cleavage is highly chemoselective and produces geminal dihalide ketones in good yields. Mechanistic investigations suggest a formation of alkyl hypoiodites from benzyl alcohols and N -iodoimides, which undergo light-induced homolytic cleavage to generate active oxygen radical species. In organic synthesis, common functionalization usually focuses on the installation or modification of functional groups without significantly changing the backbones of molecules. In stark contrast, deconstructive functionalization is attractive as it can drastically change the scaffolds of molecules to introduce new chemical space, unmask dormant functional groups, and create functionalities tethered at a predefined distance determined by ring sizes of the reactants. The carbon-carbon double bond is one of the most fundamental functionalities in organic molecules. Various methods have been developed to convert alkenes to important intermediates and fine chemical products, which play vital roles in the fields of material science, biochemistry, pharmaceutical science, and the chemical industry [1] , [2] , [3] , [4] , [5] , [6] , [7] , [8] . Deconstructive functionalization of alkenes has been well developed to introduce two functional groups at different sites of olefins (Fig. 1a ). For instance, transition-metal-catalyzed C=C bond cleavage processes, such as olefin metathesis, have found wide application in natural product and material synthesis [9] , [10] , [11] , [12] . Ozonolysis and other similar oxidations with various organic and inorganic oxidants were robust to introduce two carbonyl derivatives from a single C=C bond [13] , [14] , [15] , [16] , [17] . Aside from such well-established strategies, other types of deconstructive functionalization of alkenes producing densely functionalized scaffolds remain rare and challenging [18] , [19] , [20] , [21] , [22] , [23] , [24] , [25] , [26] , [27] . Fig. 1: Deconstructive functionalization of alkenes. a Common strategies for C=C bond cleavage. b Visible-light-mediated deconstructive oxidative geminal dihalogenation of trisubstituted alkenes (this work). DIH 1,3-diiodo-5,5-dimethyl-hydantoin, NBS N -bromosuccinimide, mCPBA meta -chloroperoxybenzoic acid. Full size image Organohalides are versatile building blocks in synthetic chemistry. They are widely utilized as precursors in transition-metal-catalyzed cross-coupling, radical reactions, nucleophilic substitutions, and metal-halide exchanges [28] , [29] , [30] . Among them, geminal dihalides represent a unique class of compounds and have been used as carbene precursors and multi-functional synthons. However, efficient synthetic pathways to synthesize geminal dihalides are quite limited, which significantly restricts the investigation and wide application of this unique family of compounds [31] , [32] , [33] , [34] , [35] . Herein, we report a direct synthetic route to geminal dihalides by photo-mediated deconstructive fragmentation of cyclic or acyclic trisubstituted alkenes (Fig. 1b ). Reaction optimization We initially designed a cascade hydrohalogenation of trisubstituted alkenes and subsequent photo-induced β -scission of the generated alcohol intermediates. Based on previous reports from groups of Chen and Zhu on photo-mediated conversion of alcohols to oxygen radicals [36] , [37] , [38] , [39] , [40] , [41] , [42] , our study commenced by using 1-phenyl-1-cyclohexene ( 1 ) as a model substrate. 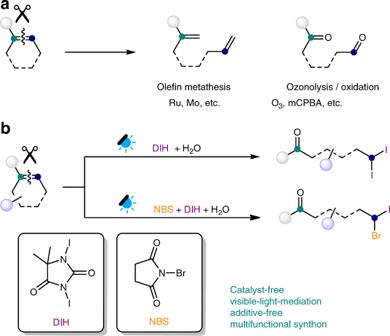Fig. 1: Deconstructive functionalization of alkenes. aCommon strategies for C=C bond cleavage.bVisible-light-mediated deconstructive oxidative geminal dihalogenation of trisubstituted alkenes (this work). DIH 1,3-diiodo-5,5-dimethyl-hydantoin, NBSN-bromosuccinimide, mCPBAmeta-chloroperoxybenzoic acid. As illustrated in Table 1 , treatment of 1 with eosin Y (1 mol%) as the photocatalyst, N -iodosuccinimide (NIS, 4 equiv), H 2 O (50 equiv) and acetoxyl benziodoxole (BIOAc, 2 equiv) in MeCN under blue light-emitting diode (LED) irradiation, the desired product, 6,6-diiodo-1-phenylhexan-1-one ( 2 ) was obtained in 40% yield (entry 1). Further investigation revealed that a similar result could be obtained in the absence of any photocatalyst (entry 2). To our surprise, 2 could be generated in 28% yield even without BIOAc (entry 3). A moderate temperature (50 °C) significantly accelerated the reaction (entries 4–5). Evaluation of solvents indicated that a mixed solvent of EtOAc/MeNO 2 (10:1) was the optimal choice, leading to the generation of 2 in 81% yield (entries 6–9). Using 1,3-diiodo-5,5-dimethyl-hydantoin (DIH) as the iodination agent afforded an improved yield compared to that with NIS (entry 10). Light irradiation was essential as no product 2 could be detected in the absence of light (entry 11). Table 1 Optimization of oxidative deconstructive geminal diiodination a . Full size table Substrate scope With the optimized conditions established, we investigated the scope of the deconstructive geminal diiodination of cyclic alkenes. As shown in Fig. 2 , a variety of aryl-substituted cyclohexene derivatives underwent deconstructive geminal diiodination effectively to deliver products 2 – 15 in moderate to good yields. Cyclohexenes containing aryl rings with electronically distinct substituents in the ortho -, meta - or para -position afforded products 2 – 10 in similar yields, with the exception of a compound bearing a strong electron-donating methoxy substituent, with which electrophilic aryl iodination occurred in the presence of DIH, resulting in a lower yield of product 5 . Various substituents on the cyclohexene ring, including methoxy, alkyl, phenyl, difluoro, were well tolerated, giving products 11 – 15 with similar yields. Naphthyl and hetero-aryl-substituted cyclohexenes were also suitable substrates, and underwent ring-opening and geminal diiodination to deliver compounds 16 – 18 with yields of 62–86%. Because the thiophene ring is very reactive towards electrophilic substitution, NIS was applied in place of DIH to avoid the iodination of the thiophene ring in the synthesis of 17 . The deconstructive geminal diiodination is not limited to cyclohexene derivatives; a range of aryl-substituted cyclopentene and cycloheptene derivatives were all viable in this deconstructive functionalization to achieve products 19 – 23 in moderate to good yields. Variation of the size of the ring containing the double bond led to geminal diiodide ketone products bearing carbon chains with varying lengths. Fig. 2: Scope of oxidative deconstructive geminal diiodination of cyclic alkenes. Isolated yields unless otherwise indicated. Performed with alkene (0.2 mmol), H 2 O (10 mmol), DIH (0.4 mmol) in EtOAc:MeNO 2 (10:1), irradiated under blue LED lamps (80 W) for 36 h at 50 °C. 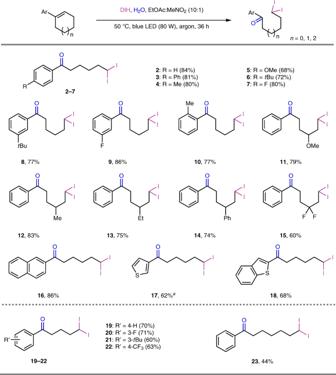Fig. 2: Scope of oxidative deconstructive geminal diiodination of cyclic alkenes. Isolated yields unless otherwise indicated. Performed with alkene (0.2 mmol), H2O (10 mmol), DIH (0.4 mmol) in EtOAc:MeNO2(10:1), irradiated under blue LED lamps (80 W) for 36 h at 50 °C.a4 equiv NIS instead of DIH. a 4 equiv NIS instead of DIH. Full size image Besides the use of DIH to generate geminal diiodo products, this strategy can be further expanded to produce potentially more useful bromo(iodo)alkanes by modifying the optimal reaction conditions by addition of NBS (Fig. 3 ). This cascade transformation was applied to a variety of aryl-substituted cyclic alkenes to afford the corresponding geminal bromo-iodination products. A variety of functional groups on the aryl rings or the cyclohexene scaffolds were well tolerated and delivered products 24 – 36 in moderate to good yields. 3,6-Dihydropyran was a good substrate for this cascade reaction thus further enriching the skeletal diversification ( 37 ). The robustness of this strategy was further explored with heteroaryl rings and cyclopentenes which generated the corresponding bromo-iodide arylketone products 38 – 40 in moderate yields. However, 1-phenyl-1-cycloheptene did not afford the corresponding bromo(iodo)alkane product 41 under our reaction conditions. Fig. 3: Scope of oxidative deconstructive geminal bromo-iodination of cyclic alkenes. Isolated yields unless otherwise indicated. Performed with alkene (0.2 mmol), NBS (0.21 mmol), H 2 O (10 mmol), DIH (0.3 mmol) in MeCN. See Supplementary Information for experimental details. a Dr values were determined by analysis of 1 H NMR spectra of the crude product mixture. Full size image As illustrated in Fig. 4a , trialkyl-substituted alkene 42 was subjected to the standard conditions for geminal diiodination and bromo-iodination, but no corresponding product could be generated. A high temperature (80 °C) could not promote geminal diiodination of 42 either, while bromo-iodination product 43 could be isolated in 21% yield. However, further increasing the temperature to 100 °C afforded only a trace amount of 43 . Control experiments (Supplementary Fig. 2 ) indicated the instability of halohydrins at high temperatures and the ineffectiveness of trialkyl-substituted halohydrins in the deconstructive iodination step. These results highlighted the importance of a suitable temperature and aromatic substituents for the success of the deconstructive geminal dihalogenation. To further expand the scope of this reaction, acyclic trisubstituted olefins were evaluated. As shown in Fig. 4b , acyclic alkenes 44 – 46 with different substituent patterns were subjected to the optimal diiodination conditions, and only the gem-alkyl-aryl-substituted olefin 46 delivered the corresponding diiodide product 47 in a useful yield (47%). Further tuning of the electronic properties in the vinyl aryl substituent ( 48 and 49 ) resulted in product 47 with similar yields. The deconstructive geminal diiodination proceeded readily with alkenes bearing different remote functionalities ( 50 and 52 ), affording products 51 and 53 , respectively, in moderate yields. Fig. 4: Investigation of other trisubstituted alkenes. a Trialkyl-substituted cyclohexenes. b Acyclic trisubstituted alkenes. Full size image Mechanistic elucidation with supporting evidence Various control experiments were performed to elucidate the reaction mechanism. First, 1 was treated with DIH or NBS and water in the absence of light to afford iodohydrin 54 or bromohydrin 55 , respectively. Tertiary alcohols 54 and 55 were subjected to the standard light-promoted conditions and afforded products 2 and 24 , respectively, but gave no product in the absence of light (Fig. 5a ). These control experiments showed that the iodohydrin and bromohydrin were intermediates in the cascade one-pot reaction. When TEMPO was added into the reaction mixture, no dihalide product could be detected, which supported a radical based reaction mechanism. ESR measurements also indicated the presence of radical species when reacting DIH with 55 in MeCN under light irradiation (Supplementary Figs. 9 and 10 ). Fig. 5: Plausible mechanism with supporting evidence. a Control experiments. b UV-Vis measurements of stoichiometry between 55 and DIH @ 450 nm. c Light on-off experiments of deconstructive geminal diiodination of 1 . d Plausible mechanism. Full size image Based on previous literatures [43] , alcohols can react with acetyl hypoiodite (AcOI) to generate alkyl hypoiodites. The O-I bonds of the alkyl hypoiodites could undergo homolytic cleavage under light irradiation to deliver a transient alkoxy radical species. We, therefore, prepared 56 by treating 55 with acetyl hypoiodite in dark, and generation of the unstable intermediate 56 was confirmed by 1 H NMR analysis of the reaction mixture (Supplementary Fig. 3 ). Irradiation of 56 formed in situ with blue LED lamps for 10 min afforded product 24 in 26% yield. When a mixture of 55 and DIH in MeCN, reacting in the dark, was examined by 1 H NMR and GC-MS analysis, 56 and 1-iodo-5,5-dimethylhydantoin were detected (Supplementary Fig. 4 – 6 ). 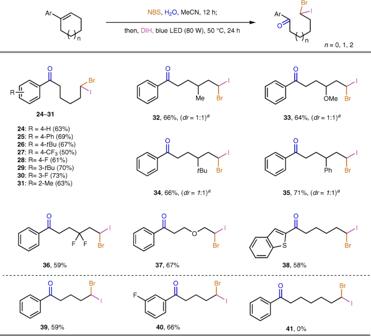Fig. 3: Scope of oxidative deconstructive geminal bromo-iodination of cyclic alkenes. Isolated yields unless otherwise indicated. Performed with alkene (0.2 mmol), NBS (0.21 mmol), H2O (10 mmol), DIH (0.3 mmol) in MeCN. See Supplementary Information for experimental details.aDrvalues were determined by analysis of1H NMR spectra of the crude product mixture. This result indicates the generation of an alkyl hypoiodite from a phenyl-substituted alcohol and DIH. Even though we cannot fully exclude the possibility of formation of an electron donor-acceptor (EDA) complex between 55 and DIH, UV-Vis measurements of different stoichiometry between 55 and DIH did not follow the curve of Job’s plot, which is normally observed for an EDA complex (Fig. 5b ). Light on/off experiments indicated that a long radical chain process is unlikely. As illustrated in Fig. 5c , the product formation ceased immediately when the light source was periodically switched off and resumed when light was turned on. Based on existing related literatures [43] , [44] , [45] , [46] , [47] and all the experimental results described above, a plausible mechanism was proposed and is described in Fig. 5d . The cascade reaction is initiated by hydroxyhalogenation of alkene I in the presence of water and an electrophilic halogen source [44] . The resulting halohydrin II reacts with DIH to deliver the alkyl hypoiodite intermediate III . Light irradiation induces the homolysis of the labile I–O bond to generate the reactive oxygen radical species IV [43] , [45] , [46] . Carbon radical V is formed by β-scission of radical IV and subsequent iodination with the iodine radical or DIH accomplishes product VI [43] , [46] , [47] , [48] , [49] , [50] , [51] . To further support the proposed ring-opening iodination, density functional theory (DFT) calculations were conducted on the model reaction of 55 with DIH. 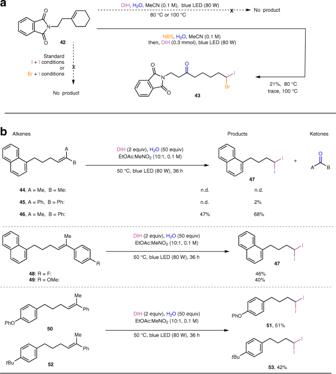Fig. 4: Investigation of other trisubstituted alkenes. aTrialkyl-substituted cyclohexenes.bAcyclic trisubstituted alkenes. The resulting energy profiles of the reaction process are displayed in Fig. 6 . The complexation of 55 and DIH leads to a zwitterionic intermediate Int1 through TS1 with active free energy of 32.6 kcal/mol. This relatively high active free energy may explain why an elevated temperature is essential for an efficient transformation (Table 1 , entry 3 vs 4). The iodine atom between the two carbonyl groups is more electrophilic than the other iodine atom in DIH, and undergoes complexation with alcohol 55 . The subsequent heterolysis of the O-I bond occurs together with the alcohol deprotonation through a transition state TS2 to give 56 and dimethyliodohydantoin with a barrier of 24.4 kcal/mol relative to Int1 . Under blue light excitation, the ground-state 56 (S 0 ) is pumped to the first singlet excited-state 56* (S 1 ) with excitation energy of 66.3 kcal/mol (2.87 eV) according to time-dependent density functional theory (TD-DFT) calculations. Homolytic cleavage of the O-I bond in 56* produces the active oxygen radical Int2 . The subsequent β -scission is a facile process with a barrier of 8.5 kcal/mol to give the transient carbon radical Int3 , followed by exergonic trapping with the iodine radical to accomplish the generation of product 24 . The geometry of the unstable alkyl hypoiodite 56 was optimized and the calculated maximum light absorption is at 432 nm (Fig. 6a ), which is close to the blue LED maximum emission (456 nm) used in this study. Fig. 6: DFT calculations for the ring-opening iodination of 55 with DIH. a Optimized geometry of 55 based on DFT calculation. b Free energy profiles for the ring-opening iodination. Full size image Further synthetic applications The oxidative geminal diiodination reaction could be achieved on gram quantities by prolonging the reaction time (Fig. 7a ). To further demonstrate the synthetic utility of our methods, derivatization of generated geminal dihalide products was attempted (Fig. 7b ). The diiodo compound 2 could be easily converted to disubstituted alkene 57 with moderate stereoselectivity by Takai-Utimoto olefination [52] , [53] . Base-promoted elimination of 2 led to vinyl iodide 58 in excellent yield with a moderate E / Z selectivity [54] . Synthetically useful geminal bis(boronate) ( 59 ) was easily produced by subjecting the diiodo compound 2 to copper-catalyzed boronation [55] . A photoredox catalyzed deiodination using Hantzsch ester as the hydrogen source reduced 2 to 60 bearing an unsubstituted alkyl chain. More interestingly, highly selective derivatization of the iodide in the bromo(iodo)alkane products could be achieved. The photoredox reaction using Hantzsch ester converted 24 to alkylbromide 61 in 90% yield. Based-promoted elimination of 24 selectively produced the corresponding vinyl bromide 62 . Bromo-iodide 24 could undergo a selective S N 2 reaction with sodium azide to afford 63 in 86% yield. Subjection of this azide ( 63 ) to copper-catalyzed azide-alkyne cycloaddition afforded a bromo triazole [56] , which could undergo further nucleophilic substitution to deliver α -functionalized triazole 64 in 69% yield. Fig. 7: Gram-scale synthesis and further synthetic diversification. a Gram-scale synthesis. b Synthetic diversification. B 2 Pin 2 bis (pinacolato)diboron, DBU 1,8-diazabicyclo (5.4.0)undec- 7-ene. Full size image In summary, we herein report a simple protocol for deconstructive geminal diiodination and bromo-iodination of trisubstituted alkenes under visible light irradiation. 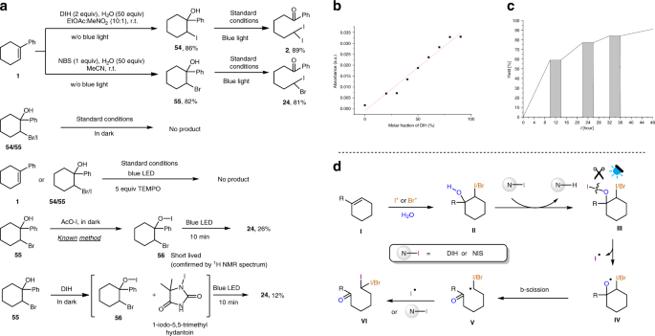Fig. 5: Plausible mechanism with supporting evidence. aControl experiments.bUV-Vis measurements of stoichiometry between55and DIH @ 450 nm.cLight on-off experiments of deconstructive geminal diiodination of1.dPlausible mechanism. The success of this transformation relies on the formation of a labile alkyl hypoiodite intermediate between the halohydrin and DIH. The protocol is distinguished by its operational simplicity, metal-free and catalyst-free characters, a wide scope of both cyclic and acyclic alkenes, delivery of useful and otherwise difficultly accessible synthons, and controllable chain length of products by choosing alkenes with different ring sizes. General procedure of the deconstructive geminal diiodination Alkene (0.2 mmol, 1 equiv) and 1,3-diiodo-5,5-dimethylhydantoin (0.4 mmol, 2 equiv), H 2 O (10 mmol, 50 equiv), and EtOAc:MeNO 2 (10:1, 2 mL) were added to a schlenk tube (10 mL) equipped with a magnetic stirring bar. Then, the reaction mixture was operated by freeze-pump-thaw procedures three times and backfilled with argon. The resulting solution was irradiated by blue LED lamps (2 × 40 W) and magnetically stirred at 50 °C. After 36 h, the reaction solution was concentrated, and the product was purified by column chromatography (SiO 2 ). The diastereomeric ratio was determined by 1 H NMR of the crude product mixture. See Supplementary Methods for details. General procedure of the deconstructive bromo-iodination Alkene (0.2 mmol) and N -bromosuccinimide (0.21 mmol, 1 equiv), H 2 O (10 mmol, 50 equiv), and MeCN (2 mL) were added to a schlenk tube (10 mL) equipped with a magnetic stirring bar. The reaction mixture was operated by freeze-pump-thaw procedures for three times and backfilled with argon. The resulting solution was magnetically stirred at 50 °C for 12 h. Then, 1,3-diiodo-5,5-dimethylhydantoin (0.3 mmol, 1.5 equiv) was added to the reaction mixture under argon. The reaction mixture was irradiated by blue LED lamps (2 × 40 W) and magnetically stirred at 50 o C. After 24 h, the reaction solution was concentrated, and the product was purified by column chromatography (SiO 2 ). The diastereomeric ratio was determined by 1 H NMR of the crude product mixture. See Supplementary Methods for details. Computational details Density functional theory (DFT) calculations were performed for the verification of the mechanism. The geometries optimization in this study (except 56 and 56* ) was performed at the (u)B3LYP‐D3(BJ) level of theory. The 6–311 + g(d,p) basis set was used for all H, C, N, and O atoms, and the Stuttgart–Dresden basis set (SDD) was employed for Br and I atoms. The nature of the stationary points (minima with no imaginary frequency or transition states with one imaginary frequency) was confirmed. The free energies of the optimized geometries were calculated at the same level of theory, taking into account the solvent effect of acetonitrile using Solvent Polarizable Continuum Model (PCM). Unless specified otherwise, the Gibbs free energy was used throughout. Considering the deviation in the free energies is ~1.89 kcal/mol from the standard state (1 atm) to 1 M in solution, we reduced by 1.89 kcal/mol to the free energy for additional steps and added by 1.89 kcal/mol for the dissociation steps [57] . For transition state, intrinsic reaction coordinate (IRC) calculations were performed to verify whether it connected with correct reactants and products or intermediates. Time-dependent density functional theory (TD-DFT) was performed to calculate the vertical excitation energies of the photodissociation process, using the CAM-B3LYP‐D3(BJ) [58] level of theory with the same basis set. 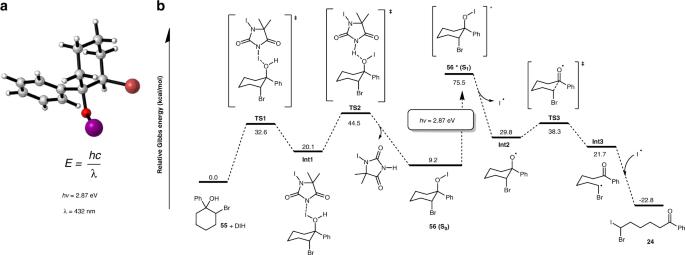Fig. 6: DFT calculations for the ring-opening iodination of 55 with DIH. aOptimized geometry of55based on DFT calculation.bFree energy profiles for the ring-opening iodination. 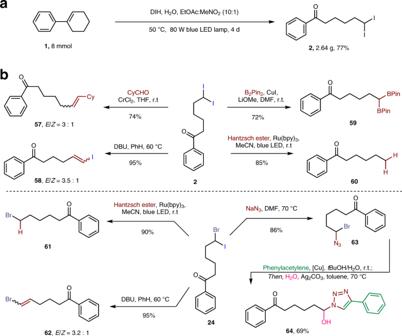Fig. 7: Gram-scale synthesis and further synthetic diversification. aGram-scale synthesis.bSynthetic diversification. B2Pin2bis (pinacolato)diboron, DBU 1,8-diazabicyclo (5.4.0)undec- 7-ene. All calculations were performed using the Gaussian 16 Rev. A.03 software suite [59] . The geometries were realized using CYLview, 1.0 [60] .